Moving from static to dynamic complexity in hydrogel design Hydrogels are water-swollen polymer networks that have been used for many decades, with applications as varied as contact lenses and super-absorbant materials. As the field of biomedical engineering has developed, hydrogels have become a prime candidate for application as molecule delivery vehicles and as carriers for cells in tissue engineering, owing to their ability to mimic many aspects of the native cellular environment (for example, high water content, mechanical properties that match soft tissues). Traditional hydrogels, formed through the covalent and non-covalent crosslinking of polymer chains, were regarded as relatively inert materials, providing a simple biomimetic three-dimensional (3D) environment, either for tissue production by local resident cells or for positioning of cells delivered in vivo . However, the simplicity of these materials may have in fact hindered their application, restricting cellular interactions with the environment and preventing uniform extracellular matrix (ECM) production and proper tissue development. In addition, these materials were limited to modelling static environments and lacked the spatiotemporal dynamic properties relevant for complex tissue processes. Fortunately, during the last decade the concepts of hydrogel design and cellular interaction have evolved, shedding light on how they may control cell behaviour, particularly for tissue engineering applications. Hydrogels with a range of mechanical properties, and capable of incorporating a wide range of biologically relevant molecules, from individual functional groups to multidomain proteins, are currently in development [1] . In addition, hydrogels are being designed with spatial heterogeneity, to either replicate properties in native tissue structures or to produce constructs with distinct regionally specific cell behavior [2] . As a result, studies to date have clearly demonstrated the possibility of creating well-defined microenvironments with control over the 3D presentation of signals to cells [3] . However, recently there has been a focus on the concept of hydrogels that exhibit dynamic complexity. These materials should evolve with time and in response to user-defined triggers or cellular behaviour. Indeed, a cadre of recent examples demonstrates that hydrogels can be used as well-defined static platforms for presenting signals to cells, and furthermore as dynamic evolving environments. It is too soon to tell how closely these materials mimic the dynamic complexity of the cell/hydrogel interface, or that of multicellular constructs or cell condensates, or to what extent dynamic hydrogels can regulate emergent biological processes such as tissue development. However, it is clear that increased material complexity is beginning to address such questions. The objective of this review is to highlight the evolution of hydrogel design towards dynamic behaviour. We first consider stable and patterned hydrogels, then hydrogels that undergo either hydrolytic or proteolytic degradation, and finally describe hydrogels with trigger-responsive properties. We particularly emphasize recent developments in hydrogel design that offer the ability to precisely control cell–microenvironment interactions, such as those found in cellular processes. We are constantly improving our understanding of biochemical and physicochemical signals in the local cellular microenvironment, and their role in cellular signalling. This has been difficult for natural materials, where many cues (for example, adhesive and mechanical) are coupled, yet synthetic hydrogels have provided a well-defined platform for experimentation. A variety of biochemical signals have been explored upon or within hydrogels, taking advantage of hydrogels as ‘blank slates’ that can be decorated with cell-interactive [4] , or growth factor-binding [5] , [6] , [7] , ligands. Hydrogels are also useful because their physical properties are biomimetic, that is, they can be designed with stiffness ranges and topographical features that are analogous to natural extracellular environments [8] . As an example, 2D polyacrylamide gels with tunable mechanical properties have provided a platform for investigating mechanotransduction behavior [9] , [10] , suggesting that stem cell fate is strongly influenced by the mechanics of the target tissue [11] . Additional related studies have emphasized the critical role of hydrogel stiffness in skeletal muscle stem cell self-renewal [12] , neural stem cell behavior [13] and megakaryocyte poiesis [14] . 3D mechanical properties are similarly important in controlling adult stem cell fate in alginate hydrogels incorporating adhesive ligands [4] . In this case, hydrogel mechanics alter the ability of a cell to cluster tethered ligands and exert tension, leading to different fate decisions (for example, adipogenic fate in softer gels and osteogenic fate in stiffer gels). Several further examples also demonstrate that 3D hydrogels support the growth of a wide variety of tissues [15] ; however, the synthesized tissue properties are often inferior to native tissue, for a range of reasons possibly related to the simplicity of these basic designs. These studies illustrate that static hydrogels are a useful, well-defined platform to efficiently probe how cell behaviour is influenced by the microenvironment, or by defined physicochemical and biological inputs. However, biological systems are rarely static and homogeneous, and there is a wealth of biology and a cadre of intriguing hypotheses to be addressed with increasing complexity in hydrogel design. Many biological processes are heterogeneous and material design is evolving to emulate them. An example of wound healing from the perspective of traditional static versus emerging hydrogels is illustrated in Fig. 1 . Wound healing is a complex process that involves spatial and temporal heterogeneity of ECM signals and is not recapitulated by static and uniform hydrogel systems. However, the complex combination of signals present in the cellular microenvironment may be mimicked by patterned hydrogel systems. Such advances allow the introduction of spatially specific cues in hydrogels, making multicellular constructs, either through co-cultures or multilineage differentiation, a possibility [16] , [17] , [18] . Spatial patterning of hydrogels also provides an additional tool for the development of high-throughput screening technology for the rapid investigation of cell–material interactions [19] , [20] , [21] , [22] . High-throughput techniques may be particularly important as cell fate is simultaneously influenced by cell–cell interactions, soluble signals, cell–ECM interactions, cell shape and mechanical forces, and natural ECMs often present cells with many distinct signals simultaneously [23] . Therefore, it is logical to expect that spatially patterned synthetic hydrogels will be needed to effectively probe the simultaneous influence of many distinct signals in order to gain meaningful biological insights or to direct cellular behaviour. 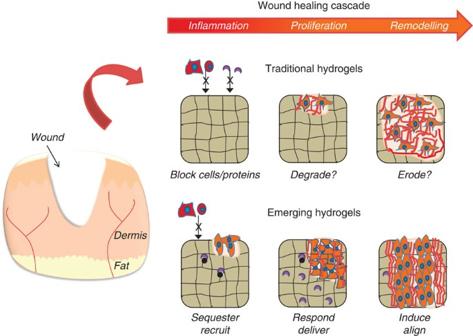Figure 1: Introducing the complexity of biological processes into hydrogels. Hydrogels are evolving from relatively inert and static materials to those incorporating sophisticated feedback mechanisms. In this theoretical example, hydrogel design is targeted to key steps in the wound healing process, where cellular recruitment, infiltration and organization can be mediated by specific cues introduced into the hydrogel design such as the ability to sequester molecules, respond to cellular signals such as degrading enzymes and organize forming tissue. Generally, hydrogels are increasing in complexity and getting better at targeting specific cascades of biochemical signals and biophysical properties. Figure 1: Introducing the complexity of biological processes into hydrogels. Hydrogels are evolving from relatively inert and static materials to those incorporating sophisticated feedback mechanisms. In this theoretical example, hydrogel design is targeted to key steps in the wound healing process, where cellular recruitment, infiltration and organization can be mediated by specific cues introduced into the hydrogel design such as the ability to sequester molecules, respond to cellular signals such as degrading enzymes and organize forming tissue. Generally, hydrogels are increasing in complexity and getting better at targeting specific cascades of biochemical signals and biophysical properties. Full size image Novel chemistry, and the application of orthogonal reactions to networks, now allows the unprecedented patterning of peptides and proteins or the alteration of network structure, even in the presence of cells. For example, multiphoton processes were used to decorate biological moieties throughout 3D systems, relying on the coupling of acrylate-modified molecules in proteolytically degradable polyethylene glycol (PEG) gels containing excess reactive groups [24] . A subsequent study illustrated the use of this technique to define regions of precise concentration and to pattern with multiple molecules throughout PEG hydrogels [25] , further expanding their complexity. In another example, orthogonal binding pairs of barnase–barstar and streptavidin–biotin were applied sequentially to pattern multiple growth factors and biological molecules ( Fig. 2 ) [26] . Specifically, one component of the pair was first immobilized into the hydrogel using two-photon chemistry and the corresponding binding partner was subsequently introduced. By applying different binding pairs in sequence, multiple factors could be immobilized. This approach follows a previously developed method where a tethered photolabile moiety was illuminated to introduce cell adhesion molecules and guide cell migration [27] . Light has also been used to introduce patterned channels that permit the migration of cells through a hydrogel [28] . 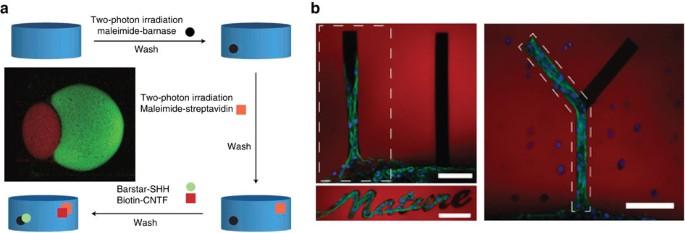Figure 2: Patterning biological cues into hydrogels. Techniques are being developed to introduce spatial control of biological cues (for example, ligands and crosslink density) into 3D hydrogels. (a) Sequential introduction of orthogonal binding pairs of barnase–barstar and streptavidin–biotin through two-photon binding of one component of the pairs (that is, barnase or streptavidin) and introduction of molecules bound to the other component (that is, barstar of biotin) to permit the coupling of multiple molecules with precise 3D patterns. Inset image illustrates this approach with fluorescent molecules. (b) Coupling of photocleavable functionality and patterning,viathe formation of gels with a click reaction, and then either patterning or photocleaving crosslinks with targeted wavelength light. Examples illustrate directed migration of fibroblasts from a fibrin clot (scale bar, 100 μm). Figure 2: Patterning biological cues into hydrogels. Techniques are being developed to introduce spatial control of biological cues (for example, ligands and crosslink density) into 3D hydrogels. ( a ) Sequential introduction of orthogonal binding pairs of barnase–barstar and streptavidin–biotin through two-photon binding of one component of the pairs (that is, barnase or streptavidin) and introduction of molecules bound to the other component (that is, barstar of biotin) to permit the coupling of multiple molecules with precise 3D patterns. Inset image illustrates this approach with fluorescent molecules. ( b ) Coupling of photocleavable functionality and patterning, via the formation of gels with a click reaction, and then either patterning or photocleaving crosslinks with targeted wavelength light. Examples illustrate directed migration of fibroblasts from a fibrin clot (scale bar, 100 μm). Full size image Other systems have been developed where orthogonal and cytocompatible click chemistry can be used to first form, and then pattern, hydrogels [29] . For example, copper-free click chemistry was used to form hydrogels around cells using the reaction of a PEG tetra-azide and a bis(DIFO3) di-functionalized polypeptide (containing a proteolytic degradable group), then an orthogonal thiol-ene photocoupling reaction was used to modify the gels with a peptide. The sequential reactions and spatial patterning permitted the gels to be controllably remodelled by cells ( Fig. 2 ). A subsequent study combined the click chemistry with a photocleavable functionality, to fabricate spatially patterned hydrogels and then to enable 3D cleavage of crosslinks [30] . Finally, a sequential crosslinking process [31] was used to pattern cell spreading and remodelling by first encapsulating cells in a hydrogel permissive to cell remodelling and then by introducing photo-induced crosslinks. The cells were unable to completely degrade the network, leading to changes in local cell spreading and subsequent stem cell differentiation. Although stable and patterned hydrogels have been very useful as a means of studying fundamental cell–material interactions, they over-simplify the complexity of the temporal dynamics present during both tissue development and repair processes. Specifically, the regulatory cascades during tissue formation and repair are extremely complex and while ‘static’ hydrogels feature some dynamic components (for example, reversible receptor–ligand binding and dynamic cell–cell interactions), little has been done to intentionally manipulate temporal properties in hydrogels, potentially owing to a lack of specific enabling technologies. However, the intrinsic properties of hydrogels lend themselves to dynamic physical and biochemical applications, including responsiveness to changes in the signalling environment. Therefore, the interface between dynamic biological systems and hydrogel material science provides an exciting area for future hydrogel design. The simplest approach to introduce temporal changes in hydrogels has been via control of hydrogel degradation, primarily to release growth factors and to eliminate the permanent implantation of a material [32] . One of the earliest examples of a degradable hydrogel features chains of poly(α-hydroxy esters), such as poly(lactic acid), incorporated at the ends of PEG molecules before the introduction of reactive groups for crosslinking [33] . Other examples include materials based on poly(vinyl alcohol) [34] , poly(propylene fumarates) [35] , dextrans [36] and hyaluronic acid [37] . In all examples, the crosslinking material changes with time, altering the physical properties and diffusivity and eventually completely degrading away ( Fig. 3 ). Likewise, non-covalently crosslinked hydrogels (for example, via ionic interactions), such as alginate, can be manipulated to alter dissociation kinetics through changes in polymer chemistry [38] . 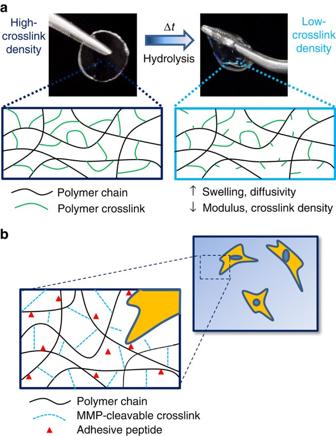Figure 3: Hydrolytically and enzymatically degradable hydrogels with properties that change with time. (a) Hydrolysis occurs relatively homogeneously throughout hydrolytically degradable hydrogels and leads to changes in the overall network crosslink density with time, which can influence properties such as diffusivity, swelling and mechanics. (b) Enzymatic degradation involves local cell-mediated proteases and is used to control cellular infiltration into the hydrogel as long as adhesive cues are also present. Figure 3: Hydrolytically and enzymatically degradable hydrogels with properties that change with time. ( a ) Hydrolysis occurs relatively homogeneously throughout hydrolytically degradable hydrogels and leads to changes in the overall network crosslink density with time, which can influence properties such as diffusivity, swelling and mechanics. ( b ) Enzymatic degradation involves local cell-mediated proteases and is used to control cellular infiltration into the hydrogel as long as adhesive cues are also present. Full size image One area in which degradation has been particularly useful is in controlling the distribution of ECM molecules by encapsulated cells [37] . In tissue engineering, it is important that these molecules are well distributed, to build up a tissue that can replicate both the form and function of native tissues. In cartilage tissue engineering approaches (with both PEG [39] and hyaluronic acid [37] hydrogels), the inclusion of fractions of hydrolytically degradable components has improved this distribution and led to improved properties, particularly functional mechanical properties. Likewise, simple hydrolytic degradation mechanisms have also hinted at the concept of dynamically influencing tissue formation via local release of ‘morphogens’ [40] , [41] . The adaptability of hydrogel synthesis allows one to introduce signalling molecules via covalent linkage, non-covalent tethering or physical entrapment [42] , or as localized depots [40] , [41] , [43] , leading to spatial morphogen gradients that mimic a common paradigm in tissue development and regeneration. Non-covalent tethering in a hydrogel can be used as a mechanism to control diffusivity of general classes of growth factors such as heparin binders [44] , or specific growth factors such as nerve growth factor [45] . In an alternative mechanism, hydrogels are also designed to be susceptible to degradation by the proteases used by cells to remodel their surroundings; specifically, peptides that may be cleaved by cell-produced proteases are incorporated into the hydrogel crosslinks [46] , [47] . A wide range of sequences were investigated that are degraded by matrix metalloproteinases (MMPs), elastases and plasmin [2] , [48] , [49] . The general susceptibility to proteases is controlled by the specific peptide sequence and there are a plethora of sequences that could be used to tailor the specific cell-mediated degradation of hydrogels ( Fig. 3 ). Generally, the hydrogels are formed by reacting a multifunctional polymer (for example, PEG macromers with vinyl sulphones or acrylates) with end groups of protease-sensitive peptides (for example, thiols from cysteine moieties), where cells and molecules can be encapsulated during gelation. The remodelling of hydrogels by cells was observed for hydrogels where both sequences for adhesion and degradation were present [50] , with degradation rates controlled by crosslink density and peptide specificity [51] . This approach has been used in numerous cases to permit cell-mediated degradation of hydrogels, leading to engineered constructs for tissues such as bone and vascular structures [49] , [52] , including examples of the incorporation of growth factors released via cellular cues [53] . Likewise, these matrices are useful as cell carriers that permit cellular morphogenesis into a variety of tissue structures [46] , [54] . Hybrid systems of synthetic and biological polymers including PEG fibrinogen [28] and hyaluronic acid [55] have also been developed with similar functionality. This approach can also be harnessed to control the delivery of molecules in diseases where protease activity is altered. Some examples of this include rheumatoid arthritis [56] , cancer [57] and after myocardial infarction [58] . In these cases, MMP levels deviate from equilibrium after injury. Thus, a system that exhibits MMP sensitivity may degrade differently depending on local MMP levels. This provides a feedback approach where local molecule delivery is regulated by cellular activity, increasing the available intricacy of release profiles. Likewise, MMP-sensitive tethers have been used for release that correlates with increased MMP activity [59] , [60] . In these cases, a pendant drug is released from matrices in response to local protease levels. These examples represent an initial foray into biological responsiveness, in the sense that hydrogels change their properties in response to a specific set of biological stimuli. Beyond purely synthetic materials, the development of protein-based materials is also becoming a possibility. In this case, molecular engineering allows for the precise introduction of a range of signal response mechanisms to control hydrogel properties (for example, via crosslinking) or cellular interactions (for example, via degradation sites) [61] . This area is likely to expand in upcoming years, as the need for the complexity found in native tissues is realized. Approaches such as directed evolution will allow the rapid assessment of sequences with specific functionality. As an alternative to covalently crosslinked structures, hydrogels may be formed via the self-assembly of peptides designed to form fibrillar structures or even to present biological signals [6] . The same cues for adhesion and degradation can be incorporated into such structures [62] , and because self-assembling hydrogels are amenable to modular design, it is possible to optimize these hydrogels for a particular outcome such as endothelialization [63] . Proteins can also be specifically engineered for added functionality and cooperativity with integrin-mediated adhesion [64] or for binding to specific molecules [5] . Finally, spatial control, as described in the previous section, may also be introduced in a dynamic fashion, providing spatiotemporal control of many hydrogel features and adding increased complexity. The use of hydrogels with either user-controlled degradation or crosslinking, or biologically responsive feedback mechanisms, highlights many novel advances in the field of hydrogel design. Moving with complexity, the field of hydrogel design is advancing past systems that change with time owing to simple hydrolysis or through cell-mediated proteolysis. Although these systems have advanced our understanding of dynamic cell–material interactions, they cannot replicate the temporal changes that occur throughout development or permit one to investigate the timed effects of specific cues on cell function. The most commonly used dynamic hydrogels to date have been designed to respond to changes in temperature and pH. For example, hydrogels composed of poly( N -isopropyl acrylamide) and poly(acrylic acid) derivatives can undergo substantial changes in volume, shape, mesh size, mechanical stiffness and optical transparency in response to temperature and/or pH. Hydrogels that include temperature-responsive or pH-responsive polymers have also been shown to dynamically vary ligand presentation to cells [65] , [66] , [67] , and to trigger the release of cells and cell sheets for tissue engineering applications [68] . These technologies have enabled proof-of-concept for new drug delivery and tissue engineering strategies; however, changes in environmental pH, temperature or ionic strength may be detrimental in some tissue engineering applications and in biological systems that typically exist under regulated homeostatic conditions. Alternatively, light is able to present precise control over temporal and spatial signals. Photoinitiated polymerizations have been widely used to form hydrogels for cell encapsulation and for the patterning of biological signals within hydrogels [69] . Light has recently been used as a trigger for the breaking of crosslinks in hydrogel networks, namely through the introduction of photosensitive o -nitro benzyl groups into the crosslinks [70] ( Fig. 4 ). This approach led to control over hydrogel structure in space and time, as well as the release of tethered signals. This synthetic system was used to probe how dynamic mechanical properties influence the phenotype of valvular interstitial cells, where changes in mechanical properties led to alterations in cell phenotype [71] . This material platform is relevant in a wide range of studies where dynamic properties are desired and is likely to push the boundaries of tunable systems. 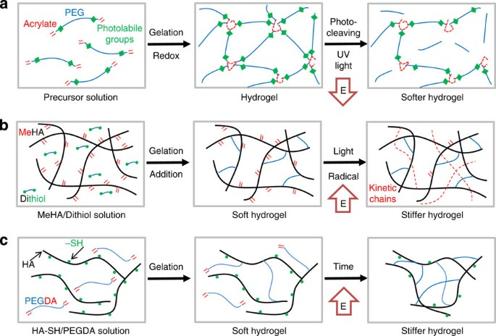Figure 4: The cleavage or introduction of crosslinks triggers changes in hydrogel properties. (a) Photocleavable groups are incorporated into PEG-based crosslinkers, and light of the appropriate wavelength cleaves crosslinks and leads to decrease in elastic modulus (E) upon exposure. (b) Two-step crosslinking process is used to first form a network and then to introduce additional crosslinks from precursors such as methacrylated hyaluronic acid (MeHA) to increase the mechanical strength in a step-wise manner. (c) Hydrogel modulus can also be increased temporally through the introduction of a crosslinker (polyethylene glycol diacrylate, PEGDA) that slowly crosslinks a modified macromolecule (for example, thiolated-hyaluronic acid, SH–HA). In this example, the kinetics and ultimate moduli can be controlled by the MW of the crosslinker. Figure 4: The cleavage or introduction of crosslinks triggers changes in hydrogel properties. ( a ) Photocleavable groups are incorporated into PEG-based crosslinkers, and light of the appropriate wavelength cleaves crosslinks and leads to decrease in elastic modulus (E) upon exposure. ( b ) Two-step crosslinking process is used to first form a network and then to introduce additional crosslinks from precursors such as methacrylated hyaluronic acid (MeHA) to increase the mechanical strength in a step-wise manner. ( c ) Hydrogel modulus can also be increased temporally through the introduction of a crosslinker (polyethylene glycol diacrylate, PEGDA) that slowly crosslinks a modified macromolecule (for example, thiolated-hyaluronic acid, SH–HA). In this example, the kinetics and ultimate moduli can be controlled by the MW of the crosslinker. Full size image Beyond degradation, there are many physiological processes where an increase in crosslinking may be of interest. For example, tissues experience increased mechanics during development and in various disease states, such as scar formation and tumour development [72] . There are only a few examples of systems where stiffness can be dynamically increased. Collagen-alginate composite hydrogels have been investigated, demonstrating mechanical properties altered by the introduction of divalent cations [73] . It is important to note that the introduction of calcium may also alter cell signalling. External stimuli such as pH can also be used to alter matrix stiffness [74] ; however, these approaches may also lead to other undesirable changes in properties such as hydrophobicity or swelling. Another class of materials involves DNA crosslinked hydrogels where the presence of free DNA may lead to increased stiffening [75] , [76] , with networks that change over a period of hours. Sequential crosslinking systems can also be used to increase hydrogel crosslinking by applying two modes of crosslinking in series [2] , varying crosslink density and in some cases susceptibility to cell-mediated degradation ( Fig. 4 ). This was recently used to probe the timing of mechanical changes on mesenchymal stem cell fate [77] . As a final example, the kinetics of gelation (crosslinking of thiolated hyaluronic acid with PEG diacrylate, Fig. 4 ) has been exploited to temporally alter substrate mechanics, mimicking changes that occur during the maturation of cardiomyocytes from mesoderm to adult myocardium [78] . Although the majority of studies to date have focused on hydrogels that respond to physicochemical stimuli (that is, light, heat and pH), emerging concepts are also focusing on hydrogels that respond to specific biological stimuli, such as protease-cleavable crosslinks within hydrogels. Beyond this, ‘biologically inspired’ mechanisms such as enzyme catalysis [79] , competitive ligand–receptor binding [80] and even nanometer-scale protein motions [81] may also be used to trigger changes in hydrogel properties ( Fig. 5 ). In some cases, these hydrogels can respond to a biological input by releasing an output, as demonstrated by insulin release in response to glucose catalysis [82] or biochemically triggered growth factor release [83] , [84] . 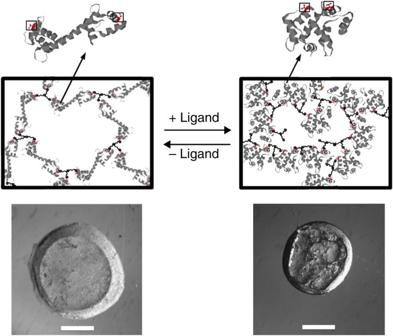Figure 5: Dynamic hydrogels that respond to biochemical inputs. Nanometer-scale biomolecule motions can be built into hydrogels to create bioresponsive hydrogels. This example (adapted from84with permission from Wiley–VCH) uses the pronounced ‘hinge motion’ of the protein calmodulin to create hydrogels that undergo programmable volume transitions in the presence of calmodulin-binding ligands (scale bar, 1 mm). Figure 5: Dynamic hydrogels that respond to biochemical inputs. Nanometer-scale biomolecule motions can be built into hydrogels to create bioresponsive hydrogels. This example (adapted from [84] with permission from Wiley–VCH) uses the pronounced ‘hinge motion’ of the protein calmodulin to create hydrogels that undergo programmable volume transitions in the presence of calmodulin-binding ligands (scale bar, 1 mm). Full size image The full potential of bioresponsive materials is becoming apparent, and is likely to become clearer in the coming decade. Bioresponsiveness may ultimately enable investigators to mimic key functions of secretory organs in the body, such as the pancreas. Importantly, they may also allow biologists and bioengineers to address new hypotheses in cell and developmental biology. Next-generation hydrogels may be designed to respond to cell-secreted biological inputs, in a manner that mimics, or even actively manipulates, the dynamics of tissue development and regeneration. Bioresponsiveness could be particularly relevant in studying and manipulating ‘emergent’ processes, such as stem cell differentiation, in which hydrogel properties that are appropriate in the early stages are likely to be dramatically different from those needed later on. For example, recent studies in standard cell culture indicate that human embryonic stem cell differentiation into spinal motor neurons [85] or cardiomyocytes [86] can be amplified by mimicking the timed soluble signalling regimen observed during early tissue development, and that the timing of signal delivery is critical. One can envision a more intelligent embodiment of this approach, in which a hydrogel responds to a change in stem cell phenotype (for example, initial lineage commitment) by changing local physical properties or by delivering a specific growth factor, thereby optimizing new tissue formation. We have only begun to develop the type of bioresponsiveness needed to manipulate tissue development in this way, and innovative synthetic strategies are critically important to expand this new area. Tissue formation processes include complex and interdependent changes in diverse environmental parameters, notably cell–ECM adhesion, cell-mediated ECM remodelling, cell–cell interaction, cell migration, soluble signalling and ECM mechanics. The complex dynamics of natural cell–ECM interactions provide both a challenge and a template for hydrogel design. Some emerging technologies in hydrogel design relate to bioinspired regulation of tissue formation, such as mimicking the ability of natural ECMs to sequester endogenous, cell-secreted signals. Sequestering can be used as a mechanism to downregulate endogenous signals that negatively impact tissue healing, such as tumour necrosis factor α (ref. 87 ). In other circumstances, sequestering may result in local amplification of signals that promote healing by ‘harnessing’ endogenous, cell-secreted growth factors [6] , [88] , [89] . Harnessing of endogenous factors may lead to a series of practical advantages when compared with delivery of purified recombinant factors. These include enhanced biological activity of native, post-translationally modified molecules, simplified paths to clinical regulatory approval and the possibility of manipulating cell–cell paracrine signalling. Interestingly, sequestering and harnessing mechanisms are also dependent on the ever-changing characteristics of the local environment, such as the concentration of cell-secreted growth factors. Therefore, hydrogels that sequester signalling molecules may soon be designed to evolve with time to optimally regulate new tissue formation. For example, it may be possible to sequester particular cytokines or growth factors during early wound healing, and then release them when needed during later stages of tissue formation. These time-dependent and environment-dependent regulatory mechanisms are common during natural wound healing, but have yet to be exploited in engineered hydrogels. Thus, as the last decade has included major advances in our ability to design complex systems, the next decade is likely to push these systems towards the complexity of biological processes and perhaps exceeding their level of control. In principle, many contemporary hydrogel synthesis schemes combine multiple dynamic, bioresponsive mechanisms into a single hydrogel. For example, glucose catalysis has led to pH-dependent hydrogel swelling and associated insulin release [90] , while protein conformational changes have led to bioresponsive changes in hydrogel swelling and associated growth factor release. The combination of these triggers would lead to unprecedented control of bioresponsiveness and molecule delivery for a specific application. The field has only begun to explore the design space of potential combinations, and the diversity of natural ECMs suggests that a wide range of dynamic functions are possible and perhaps required to achieve functional tissue engineering. In the future, we may see generic synthetic strategies to produce hydrogels that respond predictably to virtually any desired input. These systems may be used to achieve independent, dynamic regulation of multiple parameters during tissue formation and avoid the confounding effects of lurking variables, potentially via both advanced material design and high-throughput synthesis and characterization technologies. The structure of these materials may also evolve as hydrogels mimic many aspects of biological tissues, but rarely possess the hierarchical structure (for example, fibres) that provides organization and points of contact for cells. Advances in hydrogel design over the upcoming years will be made by collaboration between material scientists, bioengineers and cell biologists, and time will tell where the true utility of such advanced hydrogel systems is found. Biological complexity is partly due to cellular interactions and the dynamic nature of the local cell microenvironments, and it is not entirely clear what the level of complexity should be in the interacting hydrogel. Finally, the majority of the examples described here focused on in vitro analysis, with only a few examples of implanted hydrogels. Thus, the added complexity found in vivo needs to be addressed in the context of such materials systems. However, it is clear that such systems will allow the pursuit of questions that were unanswerable with simple static material systems and will lead to new approaches for the treatment of damaged tissues. How to cite this article: Burdick J.A. and Murphy W.L. Moving from static to dynamic complexity in hydrogel design. Nat. Commun. 3:1269 doi: 10.1038/ncomms2271 (2012).